Reduced methylation of PFKFB3 in cancer cells shunts glucose towards the pentose phosphate pathway Haem oxygenase (HO)-1/carbon monoxide (CO) protects cancer cells from oxidative stress, but the gas-responsive signalling mechanisms remain unknown. Here we show using metabolomics that CO-sensitive methylation of PFKFB3, an enzyme producing fructose 2,6-bisphosphate (F-2,6-BP), serves as a switch to activate phosphofructokinase-1, a rate-limiting glycolytic enzyme. In human leukaemia U937 cells, PFKFB3 is asymmetrically di-methylated at R131 and R134 through modification by protein arginine methyltransferase 1. HO-1 induction or CO results in reduced methylation of PFKFB3 in varied cancer cells to suppress F-2,6-BP, shifting glucose utilization from glycolysis toward the pentose phosphate pathway. Loss of PFKFB3 methylation depends on the inhibitory effects of CO on haem-containing cystathionine β-synthase (CBS). CBS modulates remethylation metabolism, and increases NADPH to supply reduced glutathione, protecting cells from oxidative stress and anti-cancer reagents. Once the methylation of PFKFB3 is reduced, the protein undergoes polyubiquitination and is degraded in the proteasome. These results suggest that the CO/CBS-dependent regulation of PFKFB3 methylation determines directional glucose utilization to ensure resistance against oxidative stress for cancer cell survival. Carbon monoxide (CO), a gas mediator generated by haem oxygenase (HO), has been shown to serve as multiple biological actions on neurovascular transmission, modulation of inflammatory responses and apoptosis via cGMP-dependent and -independent manners [1] , [2] , [3] , [4] , [5] . There is a body of evidence that HO-1 expression contributes to cancer survival, chemoresistance and tumour invasiveness in different types of cancer cells [6] , [7] , [8] , [9] , [10] , [11] . Among these studies, much attention has been paid to roles of anti-oxidative biliverdin/bilirubin and CO for protecting cancer cells, although the gas-sensitive discernible molecular mechanisms remained largely unknown. We have recently shown that physiological levels of CO exert its inhibitory action on haem-containing cystathionine β-synthase (CBS), which is the rate-limiting enzyme determining the ratio between remethylation and trans-sulphuration metabolism [4] , [12] . Since CBS can generate hydrogen sulphide (H 2 S) through the reaction utilizing cysteine and homocysteine as substrates [13] , CO-dependent inhibition of the enzyme causes H 2 S suppression and thereby plays regulatory roles for organ homeostasis [12] , [14] . Besides its role for H 2 S generation, CBS plays a role in regulating substrates for remethylation cycle including homocysteine, methionine, S-adenosylmethionine (SAM) and S-adenosylhomocysteine (SAH) [12] , [15] . CO-dependent inhibition of CBS can regulate up- and/or downregulation of protein arginine methylation through regulating cellular levels of SAM, the methyl donor, and SAH, an inhibitor of protein methyltransferases [15] , while target proteins modified by protein arginine methylation/demethylation by CO remain unknown. In clinical oncology, much attention has long been paid to CBS as a key regulator of cancer development and chemoresistance. Children with Down syndrome with acute myeloid leukaemia have significantly higher event-free survival rates compared with those with non-DS acute myeloid leukaemia. This event is linked to greater sensitivity to anti-cancer reagents and higher transcript levels of CBS as the chromosome 21-localized gene [16] . On the other hand, CBS dysfunction resulting from polymorphism induces disorders of methionine metabolism including hyperhomocysteinemia, leading to an increasing risk of head and neck cancer [17] , meningioma [18] , and colorectal adenoma and cancer [19] . Since a majority of cancer cells exhibit characteristic carbohydrate metabolism for survival such as Warburg effect [20] or mutant p53-dependent acceleration of pentose phosphate pathway (PPP) [21] , [22] , the current study aimed to mine up novel carbohydrate enzymes regulated by CO/CBS-sensitive methylation that might benefit cancer cell survival and tolerance against oxidative stress. In this study, differential metabolome/fluxome analyses of 13 C 6 -glucose utilization in cells allowed us to identify phosphofructokinase/fructose bisphosphatase type-3 (PFKFB3) as a target undergoing CO/CBS-sensitive protein arginine methylation. Arginine-methylated PFKFB3 activates glycolytic flux through increasing fructose 2,6-bisphosphate (F-2,6-BP), an allosteric activator of phosphofructokinase-1 (PFK-1) [23] , while its unmethylated form accelerates PPP that benefits NADPH/GSH system against oxidative stress. The current study provides evidence for an unexpected regulatory link from CO/CBS system towards PPP activation, serving as a mechanism for chemoresistance and anti-oxidative defence in cancer cells. CO-dependent suppression of F-2,6-BP is mediated by CBS Differences in glucose biotransformation between human monoblastic leukaemia U937 cells pretreated with 25 μM haemin for 6 h and untreated controls were examined by metabolome analysis based on capillary electrophoresis mass spectrometry (CE-MS), showing that the sum of metabolites belonging to glycolysis was decreased, while those belonging to PPP was increased significantly by HO-1 induction by haemin ( Supplementary Fig. 1 ). Under these circumstances, ATP and energy charge values were not changed by the haemin treatment. In order to determine the actual conversion of glucose to the downstream pathways, we added 13 C 6 -glucose in culture for 5 min to determine amounts of 13 C-labelled metabolic intermediates ( Fig. 1 ). The cells exhibiting HO-1 induction by the haemin treatment significantly decreased total amounts of the 13 C-labelled glycolytic metabolites (Σglycolysis), while increasing the flux towards PPP significantly, as assessed by total amounts of the 13 C-labelled PPP metabolites (Σ PPP). Such a shift from glycolysis to PPP was seen in the cells treated with CO-releasing molecule (CORM-2) for 60 min at 100 μM, showing significant increases in Xu-5P/Ru-5P and Sed-7P, and decreases in BPG and PEP in glycolytic pathway, while glucose uptake rates were unchanged ( Supplementary Fig. 2 ). 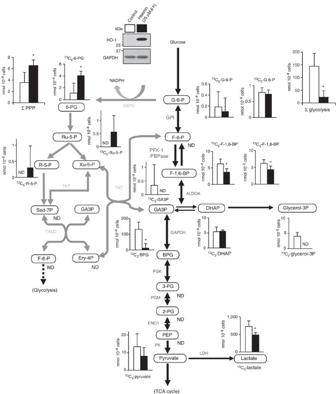Figure 1: HO-1 shifts glucose metabolism towards PPP. U937 cells were treated with 25 μM haemin for 6 h. Cells were then incubated with13C6-labelled glucose for 5 min. Data show amounts of13C-labelled metabolites in glycolysis and PPP (open bar, control; closed bar, haemin-treated cells). ∑ glycolysis; total sum values of13C6-G-6-P,13C6-F-1,6-BP,13C3-GA3P,13C3-DHAP and13C3-BPG. ∑ PPP indicates total sum values of13C6-G-6-P,13C6-6-PG,13C5-R-5-P,13C5-Ru-5-P and13C3-GA3P. BPG is expressed as total sum values of 2,3-BPG and 1,3-BPG. Inset, HO-1 expression in haemin-treated cells. Data are expressed as mean+s.d. (nmol 10−8cells) of five separate experiments. *P<0.05 versus controls (unpaired Student’st-test). ND; not detected; G-6-P, glucose 6-phosphate; F-6-P, fructose-6-phosphate; F-1,6-BP, fructose 1,6-bisphosphate; GA3P, glyceraldehyde 3-phosphate; DHAP, dihydroxyacetone phosphate; BPG, bisphosphoglycerate; 3-PG, 3-phosphoglycerate; 2-PG, 2-phosphoglycerate; PEP, phosphoenolpyruvate; 6-PG, 6-phosphogluconate; Ru-5-P, ribulose-5-phosphate; R-5-P, ribose-5-phosphate; Xu-5-P, xylulose-5-phosphate; Sed-7P, sedoheptulose-7-phosphate; Ery-4P, erythrose-4-phosphate. Figure 1: HO-1 shifts glucose metabolism towards PPP. U937 cells were treated with 25 μM haemin for 6 h. Cells were then incubated with 13 C 6 -labelled glucose for 5 min. Data show amounts of 13 C-labelled metabolites in glycolysis and PPP (open bar, control; closed bar, haemin-treated cells). ∑ glycolysis; total sum values of 13 C 6 -G-6-P, 13 C 6 -F-1,6-BP, 13 C 3 -GA3P, 13 C 3 -DHAP and 13 C 3 -BPG. ∑ PPP indicates total sum values of 13 C 6 -G-6-P, 13 C 6 -6-PG, 13 C 5 -R-5-P, 13 C 5 -Ru-5-P and 13 C 3 -GA3P. BPG is expressed as total sum values of 2,3-BPG and 1,3-BPG. Inset, HO-1 expression in haemin-treated cells. Data are expressed as mean+s.d. (nmol 10 −8 cells) of five separate experiments. * P <0.05 versus controls (unpaired Student’s t -test). ND; not detected; G-6-P, glucose 6-phosphate; F-6-P, fructose-6-phosphate; F-1,6-BP, fructose 1,6-bisphosphate; GA3P, glyceraldehyde 3-phosphate; DHAP, dihydroxyacetone phosphate; BPG, bisphosphoglycerate; 3-PG, 3-phosphoglycerate; 2-PG, 2-phosphoglycerate; PEP, phosphoenolpyruvate; 6-PG, 6-phosphogluconate; Ru-5-P, ribulose-5-phosphate; R-5-P, ribose-5-phosphate; Xu-5-P, xylulose-5-phosphate; Sed-7P, sedoheptulose-7-phosphate; Ery-4P, erythrose-4-phosphate. Full size image The results shown in Fig. 1 led us to hypothesize that HO-1 induction can inhibit the activity of PFK-1/FBPase; the hypothesis was in good agreement with increases in PPP metabolites. As expected, the PFK-1 activities in the U937 cell lysates were significantly lower in 5 μM CO-treated or haemin-treated cells than the control cells ( Fig. 2a ). PFK-1 activity is reported to be influenced by several allosteric effectors including ATP, citrate and F-2,6-BP [23] . The decreased activity of PFK-1 by CO or by HO-1 induction coincided with a decrease in F-2,6-BP, a potent allosteric activator of PFK-1 ( Fig. 2b ). The CO-treated U937 cells exhibited a time-dependent inhibition of F-2,6-BP that was insensitive to actinomycin D treatment, suggesting the inhibition process does not require de novo transcription of PFKFBs, the F-2,6-BP-generating enzymes ( Fig. 2c,d ). We also analysed mRNA expression levels of several glycolytic enzymes in U937 cells treated with or without CO treatment. No obvious differences in their expression levels were observed ( Supplementary Fig. 3 ). Since PFKFB3 and PFKFB4 constitute major isozymes in U937 leukaemia cells, effects of the isozyme knockdown were examined ( Fig. 2e ), indicating that PFKFB3 knockdown, but not PFKFB4, significantly suppressed cellular F-2,6-BP contents. 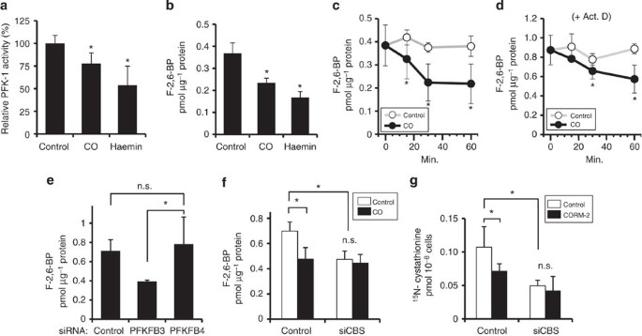Figure 2: CO suppresses PFK-1 activity by downregulation of F-2,6-BP levels in U937 cells. (a) Suppression of PFK-1 activities in U937 cell lysates by CO or by haemin. Data indicate mean+s.d. of four separate sets of experiments. *P<0.05 versus controls (ANOVA with Fischer’s multiple comparison test). (b) Suppression of F-2,6-BP contents by CO or haemin. Data indicate mean+s.d. of four separate experiments. *P<0.05 versus controls (ANOVA with Fischer’s multiple comparison test). (c,d) indicate suppression of F-2,6-BP contents after exposure to CO in the absence (c) or presence (d) of actinomycin D (Act.D). Open and closed circles indicate data from the control and those from the CO-exposing group, respectively. Data represent mean±s.d. of four separate experiments. *P<0.05 versus controls at each time points (unpaired Student’st-test). (e) Specific inhibitory action of siPFKFB3, but not of siPFKFB4, on F-2,6-BP contents. Data indicate mean+s.d. of four separate experiments. *P<0.05 between PFKFB3 knockdown and PFKFB4 knockdown. n.s.; not significant (ANOVA with Fischer’s multiple comparison test). (f) Cancellation of CO-induced suppression of F-2,6-BP by CBS knockdown. Open and closed bars indicate data in the absence or presence of 5 μM CO. Data show the mean+s.d. of five independent experiments. *P<0.05 versus controls (ANOVA with Fischer’s multiple comparison test). (g) Disappearance of CORM-induced suppression of flux into trans-sulphuration by CBS knockdown. U937 cells were treated with 100 μM RuCl3(negative control, open bars) or 100 μM CORM-2 (filled bars) for 1 h, and then incubated with15N-labelled methionine for 5 min. Graph shows the amount of15N-cystathionine. Data show the mean+s.d. of four independent experiments. *P<0.05 versus controls (ANOVA with Fischer’s multiple comparison test). Procedures for treatment with CO at 5 μM for 30 min or with haemin at 25 μM for 6 h were identical throughout (a–f). n.s., not significant. Figure 2: CO suppresses PFK-1 activity by downregulation of F-2,6-BP levels in U937 cells. ( a ) Suppression of PFK-1 activities in U937 cell lysates by CO or by haemin. Data indicate mean+s.d. of four separate sets of experiments. * P <0.05 versus controls (ANOVA with Fischer’s multiple comparison test). ( b ) Suppression of F-2,6-BP contents by CO or haemin. Data indicate mean+s.d. of four separate experiments. * P <0.05 versus controls (ANOVA with Fischer’s multiple comparison test). ( c , d ) indicate suppression of F-2,6-BP contents after exposure to CO in the absence ( c ) or presence ( d ) of actinomycin D (Act.D). Open and closed circles indicate data from the control and those from the CO-exposing group, respectively. Data represent mean±s.d. of four separate experiments. * P <0.05 versus controls at each time points (unpaired Student’s t -test). ( e ) Specific inhibitory action of siPFKFB3, but not of siPFKFB4, on F-2,6-BP contents. Data indicate mean+s.d. of four separate experiments. * P <0.05 between PFKFB3 knockdown and PFKFB4 knockdown. n.s. ; not significant (ANOVA with Fischer’s multiple comparison test). ( f ) Cancellation of CO-induced suppression of F-2,6-BP by CBS knockdown. Open and closed bars indicate data in the absence or presence of 5 μM CO. Data show the mean+s.d. of five independent experiments. * P <0.05 versus controls (ANOVA with Fischer’s multiple comparison test). ( g ) Disappearance of CORM-induced suppression of flux into trans-sulphuration by CBS knockdown. U937 cells were treated with 100 μM RuCl 3 (negative control, open bars) or 100 μM CORM-2 (filled bars) for 1 h, and then incubated with 15 N-labelled methionine for 5 min. Graph shows the amount of 15 N-cystathionine. Data show the mean+s.d. of four independent experiments. * P <0.05 versus controls (ANOVA with Fischer’s multiple comparison test). Procedures for treatment with CO at 5 μM for 30 min or with haemin at 25 μM for 6 h were identical throughout ( a – f ). n.s., not significant. Full size image As mentioned in the Introduction section, CBS is a CO-sensitive key enzyme that regulates protein arginine methylation [15] , leading us to examine whether the CO/CBS system is involved in mechanisms for CO-sensitive downregulation of F-2,6-BP in the cell. As seen in Fig. 2f , CBS knockdown by siRNA significantly suppressed basal F-2,6-BP contents in the same cells. Such cells rendered insensitive to the same concentration of CO. We next examined whether CO suppresses trans-sulphuration via CBS inhibition. As expected, the CO treatment significantly inhibited intracellular conversion of 15 N-labelled methionine to 15 N-cystathionine by CBS. This result is in good agreement with our previous studies in vivo [12] . Furthermore, the CBS-knocked down cells suppressed the basal flux for the cystathionine generation, and became insensitive to the CO application ( Fig. 2g ). Collectively, these results raised a possibility that CO modulates glucose biotransformation through post-translational mechanisms involving arginine methylation of PFKFB3 in the cells. PRMT1 contributes to protein arginine methylation of PFKFB3 We found that human PFKFB3 possessed two RXR(R) motifs, presumably recognized by protein arginine methyltransferase 1 (PRMT1) [24] in the primary structure ( Supplementary Fig. 4 ). The fact led us to examine whether the enzyme modification by arginine methylation is involved in mechanisms for attenuating F-2,6-BP levels through the CO/CBS pathway. To test this hypothesis, arginine methylation of PFKFB3 was detected in vitro by the incorporation of [ 3 H]-methyl group derived from [ 3 H]-SAM with autoradiography ( Fig. 3a ). Among different PRMT isozymes, PRMT1 and PRMT4 can transfer methyl group towards GST-tagged PFKFB3. In order to identify the residues of arginine methylation, three human PFKFB3 fragments including full-length (1–520), N-terminal (1–246) and C-terminal (247–520) were constructed, since the latter two fragments contain a single RXRR (131-RERR-134) or RXR (443-RER-445) domain, respectively ( Fig. 3b ). In vitro methylation assay in the presence of PRMT1 or 4 and the radioactive SAM with each PFKFB3 fragments showed that PRMT1 and PRMT4 appeared to be responsible for dimethylation at 131-RERR-134 domain of the N-terminal fragment of PFKFB3 in vitro ( Fig. 3c ). Among three arginine residues in the N-terminal fragment, R131 and R134, but not R133, serve as critical sites of PFKFB3 dimethylation by PRMT1, so far as judged by results of site-directed mutagenesis assay of in vitro methylation assay in the presence of PRMT1, a major asymmetric methyltransferase [24] ; replacement with either R131K or R134K partially suppressed, and the double mutants R131/134K completely abolished the PRMT1-dependent methylation signals ( Fig. 3d ). 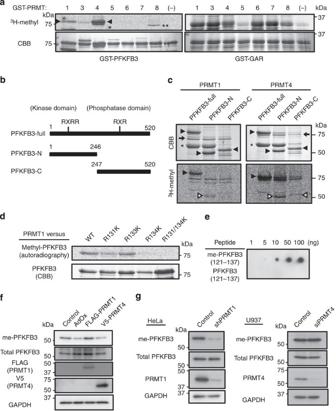Figure 3: PRMT1 is responsible for site-specific protein arginine methylation of PFKFB3in vitro. (a)In vitromethylation assays of GST-fused recombinant human PFKFB3 in the presence of PRMT isoforms (PRMT1,3-8). Methylation of PFKFB3 was detected by the incorporation of [3H]-methyl group derived from [3H]-SAM with autoradiography. Right lanes indicate data showing arginine methylation of GST-fused GAR (glycine and arginine rich) domain in human fibrillarin as a positive control, indicating that all isoforms used in this assay are functionally intact. Note that PRMT1 specifically methylates GST-PFKFB3 (arrowhead), while PRMT4 not only methylates GST-PFKFB3 (arrowhead) but also induces self-methylation (single asterisk in lane 4 in the left set). Double asterisks (**) indicate self-methylation of PRMT8. (b) The schematic diagram of human PFKFB3 fragments including full-length (1–520), N-term (1–246) and C-term (247–520). (c) Site-specific arginine methylation of GST-PFKFB3 by PRMT1. Closed arrowheads indicate the bands derived from the fragments of GST-PFKFB3. Arrows indicate GST-PRMT1 and 4. Open arrowheads indicate the methylated fragments of truncated PFKFB3. Asterisks indicate a non-specific band. (d) Identification of critical arginine residues for PFKFB3 methylation. R131 and R134 serve as critical sites of PFKFB3 methylation by PRMT1. In this assay, total amounts of substrates were analysed by Coomassie Brilliant Blue staining. (e) Dot blot analysis of non-methyl and dimethyl-peptide (R131/134) from human PFKFB3 (121-137) with the anti-dimethyl-PFKFB3 (R131/134) antibody, indicating dose-dependent signals without reacting with the unmethylated enzyme. (f) PRMT1, but not PRMT4 activates R131/134 arginine methylation of PFKFB3 in cultured cells. HEK293 cells were treated with or without AdOx for demethylation for 16 h, and then transfected with FLAG-PRMT1 or V5-PRMT4. (g) Effects of PRMT1 or PRMT4 knockdown on dimethylation of PFKFB3 in cancer cells. PRMT1 knockdown by shPRMT1 suppressed methylation of PFKFB3, while PRMT4 knockdown by siPRMT4 was unable to suppress R131/134 methylation status of PFKFB3 (HeLa cells and U937 cells). Lysates were immunoblotted with anti-dimethyl-PFKFB3 (R131/134), anti-PFKFB3, anti-FLAG, anti-V5, anti-PRMT1, anti-PRMT4 and anti-GAPDH antibodies. Figure 3: PRMT1 is responsible for site-specific protein arginine methylation of PFKFB3 in vitro . ( a ) In vitro methylation assays of GST-fused recombinant human PFKFB3 in the presence of PRMT isoforms (PRMT1,3-8). Methylation of PFKFB3 was detected by the incorporation of [ 3 H]-methyl group derived from [ 3 H]-SAM with autoradiography. Right lanes indicate data showing arginine methylation of GST-fused GAR (glycine and arginine rich) domain in human fibrillarin as a positive control, indicating that all isoforms used in this assay are functionally intact. Note that PRMT1 specifically methylates GST-PFKFB3 (arrowhead), while PRMT4 not only methylates GST-PFKFB3 (arrowhead) but also induces self-methylation (single asterisk in lane 4 in the left set). Double asterisks (**) indicate self-methylation of PRMT8. ( b ) The schematic diagram of human PFKFB3 fragments including full-length (1–520), N-term (1–246) and C-term (247–520). ( c ) Site-specific arginine methylation of GST-PFKFB3 by PRMT1. Closed arrowheads indicate the bands derived from the fragments of GST-PFKFB3. Arrows indicate GST-PRMT1 and 4. Open arrowheads indicate the methylated fragments of truncated PFKFB3. Asterisks indicate a non-specific band. ( d ) Identification of critical arginine residues for PFKFB3 methylation. R131 and R134 serve as critical sites of PFKFB3 methylation by PRMT1. In this assay, total amounts of substrates were analysed by Coomassie Brilliant Blue staining. ( e ) Dot blot analysis of non-methyl and dimethyl-peptide (R131/134) from human PFKFB3 (121-137) with the anti-dimethyl-PFKFB3 (R131/134) antibody, indicating dose-dependent signals without reacting with the unmethylated enzyme. ( f ) PRMT1, but not PRMT4 activates R131/134 arginine methylation of PFKFB3 in cultured cells. HEK293 cells were treated with or without AdOx for demethylation for 16 h, and then transfected with FLAG-PRMT1 or V5-PRMT4. ( g ) Effects of PRMT1 or PRMT4 knockdown on dimethylation of PFKFB3 in cancer cells. PRMT1 knockdown by shPRMT1 suppressed methylation of PFKFB3, while PRMT4 knockdown by siPRMT4 was unable to suppress R131/134 methylation status of PFKFB3 (HeLa cells and U937 cells). Lysates were immunoblotted with anti-dimethyl-PFKFB3 (R131/134), anti-PFKFB3, anti-FLAG, anti-V5, anti-PRMT1, anti-PRMT4 and anti-GAPDH antibodies. Full size image To address PFKFB3 methylation at R131/R134 in vivo , we raised the polyclonal antibody against asymmetric di-methylated PFKFB3 peptide (121–137). The newly generated antibody could detect the asymmetrically di-methylated peptide in a dose-dependent manner without reacting to non-methylated PFKFB3 peptide ( Fig. 3e ). We then examined whether alterations in PRMT1 expression in cells can regulate levels of methylated and unmethylated PFKFB3 ( Fig. 3f ). To be noted was the fact that di-methylated PFKFB3 occurs in the untreated control cells, while the constitutive levels of dimethylation is suppressed by the adenosine dialdehyde (AdOx) treatment ( Fig. 3f ). Overexpression of PRMT1, but not that of PRMT4, in the AdOx-pretreated cells increased amounts of di-methylated PFKFB3. Furthermore, while the cells undergoing knockdown by shPRMT1, but not by siPRMT4, abolished methylated PFKFB3 almost completely ( Fig. 3g ). These results suggest that PRMT1, but not PRMT4, is responsible for site-specific dimethylarginine modification of PFKFB3 at R131 and R134 in cells. CO modulates PFKFB3 methylation to be polyubiquitinated Using the polyclonal antibody recognition of di-methylated PFKFB3 (R131/134), we examined if the haem-degrading catalytic activity of HO-1 is necessary to regulate post-translational arginine methylation of PFKFB3 ( Fig. 4 ). Constitutively expressed methyl-PFKFB3 in control U937 cells was suppressed by HO-1 induction elicited by haemin ( Fig. 4a ). To be noted was the fact that a stable gene transfectant of wild-type (WT) HO-1 caused disappearance of methylated PFKFB3 that coincided with notable downregulation of total PFKFB3 amounts in the cells ( Fig. 4b ). On the other hand, the transfectant of mutant HO-1 (H25A), which is unable to catalyse haem because it lacks the histidine residue for the axial haem ligand and thereby serves as a dominant negative for the cellular catalytic activity of HO-1 (ref. 25 ), exhibited robust elevation of the methylated enzyme. Under these circumstances, total amounts of PFKFB3 were also maintained ( Fig. 4b ). Surprisingly, in these HO-1 expression lines, no differences in PFKFB3 mRNA expression level were observed ( Supplementary Fig. 3b ). Furthermore, in the WT-HO-1-transfected cells, treatment with chromium mesoprotoporphyrin (CrMP), a potent HO inhibitor, increased amounts of methylated PFKFB3 in a dose-dependent manner, suggesting the catalytic activity of HO-1 is necessary to decrease methylated PFKFB3 ( Fig. 4c ). Exposure of CO at the physiologically relevant concentration (5 μM) to U937 cells reproduced time-dependent decreases in methylated PFKFB3. Of importance was the observation that CBS knockdown decreased the basal amounts of methylated PFKFB3 and rendered the cells less sensitive to the CO exposure ( Fig. 4d ). Similar results were observed in HEK293 cells expressing shCBS ( Supplementary Fig. 5 ). 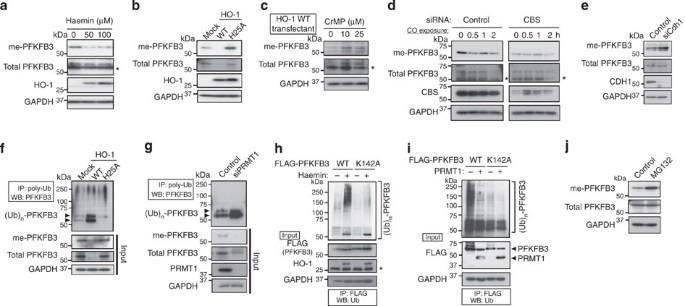Figure 4: HO-1/CO triggers K142 polyubiquitination of PFKFB3. (a) Demethylation of PFKFB3 in U937 cells treated with haemin for 6 h. (b) Alterations in arginine methylation status of PFKFB3 in U937 cells stably transfected with WT and mutant (H25A) HO-1 that lacks in catalytic activity. Note that transfection with WT but not with H25A mutant HO-1 causes PFKFB3 demethylation. Lysates were analysed by western blotting with anti-dimethyl-PFKFB3, anti-PFKFB3 and anti-HO-1 antibodies. (c) Effects of CrMP, an HO inhibitor of methylation of PFKFB3, indicating that the catalytic activity of HO is necessary for PFKFB3 demethylation. (d) Temporal alterations in methylation of PFKFB3 in U937 cells transfected with siRNA (control or siCBS) exposed to 5 μM CO. Lysates were analysed by western blotting using anti-dimethyl-PFKFB3, anti-PFKFB3 and anti-CBS antibodies. In the right panels, note suppression of basal me-PFKFB3 signals and disappearance of the CO-induced signal inhibition in siCBS-transfected cells. (e) Effects of Cdh1-silencing in HeLa cells on R131/134 methylation of PFKFB3. Note that knockdown of Cdh1 increases methylated PFKFB3. (f) Role of HO-1 catalytic activities in the regulation of demethylation and polyubiquitination of PFKFB3. PFKFB3 endogenous polyubiquitination ((Ub)n-PFKFB3) was observed by WT, but not by H25A mutant HO-1 transfection. (g) Effects of PRMT1 knockdown on PFKFB3 polyubiquitination. U937 cells were transfected with siRNA against control (scramble) or against PRMT1. Lysates were immunoprecipitated with anti-polyubiquitin antibody. The eluates are analysed with anti-PFKFB3 antibody. Lysates for input were immunoblotted with anti-dimethyl-PFKFB3 (R131/134), anti-PFKFB3 and anti-PRMT1. The expression level of GAPDH is used as a loading control. (h) Roles of K142 in HO-1-triggered PFKFB3 polyubiquitination. (i) Roles of K142 in PRMT1-sensitive PFKFB3 polyubiquitination. Note that K142A mutant transfectants are insensitive to HO-1 induction or to PRMT1 overexpression. Lysates were immunoprecipitated with anti-FLAG antibody. The eluates are analysed with anti-ubiquitin antibody. The expression level of GAPDH is used as a loading control. (j) Effects of MG132, a proteasomal inhibitor, on arginine dimethylation of PFKFB3. MG132 (10 μM) was treated for 6 h. All data are representative of at least two separate experiments. Asterisks in (a,c,d,h) indicate non-specific bands resulting from the polyclonal antibody. Figure 4: HO-1/CO triggers K142 polyubiquitination of PFKFB3. ( a ) Demethylation of PFKFB3 in U937 cells treated with haemin for 6 h. ( b ) Alterations in arginine methylation status of PFKFB3 in U937 cells stably transfected with WT and mutant (H25A) HO-1 that lacks in catalytic activity. Note that transfection with WT but not with H25A mutant HO-1 causes PFKFB3 demethylation. Lysates were analysed by western blotting with anti-dimethyl-PFKFB3, anti-PFKFB3 and anti-HO-1 antibodies. ( c ) Effects of CrMP, an HO inhibitor of methylation of PFKFB3, indicating that the catalytic activity of HO is necessary for PFKFB3 demethylation. ( d ) Temporal alterations in methylation of PFKFB3 in U937 cells transfected with siRNA (control or siCBS) exposed to 5 μM CO. Lysates were analysed by western blotting using anti-dimethyl-PFKFB3, anti-PFKFB3 and anti-CBS antibodies. In the right panels, note suppression of basal me-PFKFB3 signals and disappearance of the CO-induced signal inhibition in siCBS-transfected cells. ( e ) Effects of Cdh1-silencing in HeLa cells on R131/134 methylation of PFKFB3. Note that knockdown of Cdh1 increases methylated PFKFB3. ( f ) Role of HO-1 catalytic activities in the regulation of demethylation and polyubiquitination of PFKFB3. PFKFB3 endogenous polyubiquitination ((Ub) n -PFKFB3) was observed by WT, but not by H25A mutant HO-1 transfection. ( g ) Effects of PRMT1 knockdown on PFKFB3 polyubiquitination. U937 cells were transfected with siRNA against control (scramble) or against PRMT1. Lysates were immunoprecipitated with anti-polyubiquitin antibody. The eluates are analysed with anti-PFKFB3 antibody. Lysates for input were immunoblotted with anti-dimethyl-PFKFB3 (R131/134), anti-PFKFB3 and anti-PRMT1. The expression level of GAPDH is used as a loading control. ( h ) Roles of K142 in HO-1-triggered PFKFB3 polyubiquitination. ( i ) Roles of K142 in PRMT1-sensitive PFKFB3 polyubiquitination. Note that K142A mutant transfectants are insensitive to HO-1 induction or to PRMT1 overexpression. Lysates were immunoprecipitated with anti-FLAG antibody. The eluates are analysed with anti-ubiquitin antibody. The expression level of GAPDH is used as a loading control. ( j ) Effects of MG132, a proteasomal inhibitor, on arginine dimethylation of PFKFB3. MG132 (10 μM) was treated for 6 h. All data are representative of at least two separate experiments. Asterisks in ( a , c , d , h ) indicate non-specific bands resulting from the polyclonal antibody. Full size image Observation that stable transfection of enzymatically intact WT-HO-1 caused downregulation of methylated PFKFB3 led us to hypothesize that, once being unmethylated by HO-1/CO, the enzyme becomes sensitive to polyubiquitination and proteosomal degradation. A recent study demonstrated that PFKFB3 is suffering from constant proteasome degradation through the polyubiquitination on K142 residue in rat neuron [26] . The crystal structure of PFKFB3 reveals that arginine residues (R131/134) for dimethylation by PRMT1 are closely located to lysine (K142) for ubiquitination on the same helix ( Supplementary Fig. 6 ), suggesting that arginine dimethylaton of PFKFB3 might affect the ubiquitination level of K142 and the stability of the enzyme. Actually, knocking down Cdh1, a cofactor for polyubiquitination ((Ub) n ) [26] , notably increased methylated PFKFB3 without altering total PFKFB3 in HeLa cells ( Fig. 4e ), suggesting roles of the polyubiquitination process in regulating methylated PFKFB3. Using the U937 cell lysates, we immunoprecipitated polyubiquitinated PFKFB3 ((Ub) n -PFKFB3 in Fig. 4f,g ) by the anti-poly-Ub antibody and served as samples for western blot by the anti-PFKFB3 antibody, indicating that overexpression of WT HO-1, but not that of H25A mutant, caused a notable increase in (Ub) n -PFKFB3 (arrowheads in Fig. 4f ). In addition, knocking down PRMT1 by siPRMT1 caused an increase in (Ub)n-PFKFB3 ( Fig. 4g ). We were unable to show polyubiquitinated PFKFB3, indicating varied molecular sizes of the polyubiquitinated enzymes, because sensitive antibodies suitable for the analyses were unavailable. Therefore, HEK293 cells overexpressing FLAG-tagged WT PFKFB3 or K142 mutant PFKFB3 were prepared; these cells enabled us to detected polyubiquitinated proteins by the anti-ubiquitin antibody under stimulation with HO-1 induction or with PRMT1 overexpression as methylation-switching procedures, respectively. As seen, HO-1 induction by haemin in WT-PFKFB3-transfected cells notably displayed formation of polyubiquitinated PFKFB3 proteins with different molecular sizes ( Fig. 4h ). On the other hand, PRMT1-overexpressing cells exhibited downregulation of polyubiquitinated PFKFB3 ( Fig. 4i ). In both experiments, K142A mutant PFKFB3 did not undergo polyubiquitination in response to the HO-1 induction or to PRMT1 overexpression in U937 cells. These results collectively suggested that the methylation switch determines PFKFB3 ubiquitination at K142. Finally, MG132, a proteosomal inhibitor, increased basal amounts of methylated PFKFB3 with total PFKFB3 being unchanged ( Fig. 4j ). Although the relationship between proteosomal degradation and fates of PFKFB3 methylation should be further examined, these results suggest that R131/134-unmethylated form of PFKFB3 serves as a target of polyubiquitination at K142, and that HO-1/CO accelerates this process. CO modulates PFKFB3 methylation to protect from oxidants As a result of the decrease in F-2,6-BP generation by decreased PFKFB3 methylation, U937 cells exposed to CO or to HO-1 induction by haemin exhibited significant elevation of cellular amounts of NADPH that coincided with an increasing NADPH/NADP + ratio ( Fig. 5a ). U937 cells exposed to CO or those pretreated with haemin became significantly resistant to H 2 O 2 ( Fig. 5b ). Since CO exposure as well as the HO-1 induction decreased amounts of trans-sulphuration metabolites via CO-dependent CBS inhibition [12] , [15] , total amounts of reduced and oxidized glutathione (GSH+2GSSG) were modestly suppressed in U937 cells. Even under such circumstances, the ratio between GSH and GSSG was significantly increased in the CO-treated cells, suggesting that anti-oxidative capacity of the cell was potentiated ( Fig. 5c ). Moreover, the cells transfected with siCBS or siPRMT1 exhibited lesser sensitivity to H 2 O 2 that coincided with increased NADPH contents ( Supplementary Fig. 7 ). In the same cells, we examined effects of the CBS knockdown by siRNA on cisplatin sensitivity. CBS knockdown caused a decrease in methylated PFKFB3 in the cells ( Fig. 5d ), and acquired chemoresistance against cisplatin [27] ( Fig. 5e ). 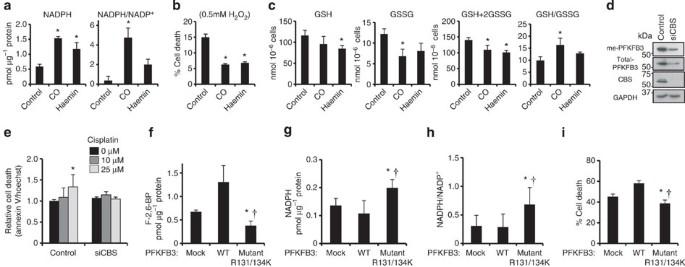Figure 5: Protective effects of CO on oxidative cell injury through enhancing NADPH–glutathione system in U937 cells. (a) Intracellular NADPH levels and NADPH/NADP+ratio in U937 cells treated with CO or with haemin. Data indicate mean+s.d. (n=4–6). *P<0.05 versus controls. (b) Inhibitory effect of CO or haemin on H2O2-induced cell death. Cells were exposed to 0.5 mM H2O2for 1 h. Data indicate mean+s.d. of four separate experiments *P<0.05 versus controls. (c) Alterations in reduced and oxidized glutathione levels in U937 cells treated with CO and haemin. Data indicate mean+s.d. (n=5–8). *P<0.05 versus controls. Procedures for treatment with CO at 5 μM for 30 min or with haemin at 25 μM for 6 h were identical throughout experiments. (d) The blot shows the methylation status of PFKFB3 in U937 cells transfected with siCBS. The expression level of GAPDH is used as a loading control. (e) Effect of CBS knockdown on cisplatin-induced apoptosis in U937 cells. U937 cells were treated with increasing concentrations of cisplatin for 6 hours. Cell viability was determined as fluorescence signal derived from annexin V-FITC in the apoptotic cells. Data indicate the values of relative cell death as means+s.d. of four separate experiments. *P<0.05 versus control without cisplatin treatment. Panels (f–i): Effects of overexpression of WT-PFKFB3 or mutant R131/134K-PFKFB3 on redox metabolites in HEK293 cells. (f) F-2,6-BP contents, (g) NADPH contents, (h) NADPH/NADP+ratio and (i) sensitivity to H2O2. In these experiments, HEK293 cells were transfected with mock, WT or nonmethylable mutant (R131/134K) PFKFB3. Data indicate mean+s.d. of five separate experiments. *P<0.05 (mock versus R131/134K),†P<0.05 (WT versus R131/134K). ANOVA with Fischer’s multiple comparison test was used for determining statistical significance throughout this figure. Figure 5: Protective effects of CO on oxidative cell injury through enhancing NADPH–glutathione system in U937 cells. ( a ) Intracellular NADPH levels and NADPH/NADP + ratio in U937 cells treated with CO or with haemin. Data indicate mean+s.d. ( n =4–6). * P <0.05 versus controls. ( b ) Inhibitory effect of CO or haemin on H 2 O 2 -induced cell death. Cells were exposed to 0.5 mM H 2 O 2 for 1 h. Data indicate mean+s.d. of four separate experiments * P <0.05 versus controls. ( c ) Alterations in reduced and oxidized glutathione levels in U937 cells treated with CO and haemin. Data indicate mean+s.d. ( n =5–8). * P <0.05 versus controls. Procedures for treatment with CO at 5 μM for 30 min or with haemin at 25 μM for 6 h were identical throughout experiments. ( d ) The blot shows the methylation status of PFKFB3 in U937 cells transfected with siCBS. The expression level of GAPDH is used as a loading control. ( e ) Effect of CBS knockdown on cisplatin-induced apoptosis in U937 cells. U937 cells were treated with increasing concentrations of cisplatin for 6 hours. Cell viability was determined as fluorescence signal derived from annexin V-FITC in the apoptotic cells. Data indicate the values of relative cell death as means+s.d. of four separate experiments. * P <0.05 versus control without cisplatin treatment. Panels ( f – i ): Effects of overexpression of WT-PFKFB3 or mutant R131/134K-PFKFB3 on redox metabolites in HEK293 cells. ( f ) F-2,6-BP contents, ( g ) NADPH contents, ( h ) NADPH/NADP + ratio and ( i ) sensitivity to H 2 O 2 . In these experiments, HEK293 cells were transfected with mock, WT or nonmethylable mutant (R131/134K) PFKFB3. Data indicate mean+s.d. of five separate experiments. * P <0.05 (mock versus R131/134K), † P <0.05 (WT versus R131/134K). ANOVA with Fischer’s multiple comparison test was used for determining statistical significance throughout this figure. Full size image Using HEK293 cells, which enabled us to prepare stable transfectants easily, we examined effects of exogenously introduced WT-PFKFB3 and the unmethylable R131/134K mutant. As seen, the WT-transfectant increased, and the R131/134K mutant transfectant decreased basal contents of F-2,6-BP versus the mock transfectant ( Fig. 5f ). Moreover, transfection of PRMT1, but not that of PRMT4, increased F-2,6-BP contents in WT-PFKFB3-expressing cells. By contrast, the R131/134K mutant exhibited significantly lower contents of F-2,6-BP, and did not increase them in response to PRMT1 overexpression ( Supplementary Fig. 8 ). The cells overexpressing the R131/134K mutant significantly increased cellular amounts of NADPH and the NADPH/NADP + ratio than mock and WT transfectants ( Fig. 5g,h ). Under these circumstances, the cells overexpressing R131/134K mutant PFKFB3 exhibited lesser susceptibility against H 2 O 2 than those of mock or WT transfectants ( Fig. 5i ), showing dominant negative effects of the mutant. These results collectively suggested that the R131/134-unmethylated form of PFKFB3 is crucial for supporting cellular NADPH against oxidative stress. As shown in structure of PFKFB3 monomer ( Supplementary Fig. 6 ), positively charged R131/134 residues might strengthen fructose-6-phosphate (F-6-P) binding to R133 as their proximal residue. To examine whether an unmethylable and uncharged mutant of PFKFB3, which weakens F-6-P binding to R133, might facilitate a shift of glucose metabolism from glycolysis to PPP to upregulate NADPH, we established HEK293 cells overexpressing the R131/134K or R131/134L mutant PFKFB3, and compared the 13 C 6 -glucose fluxes versus the cells overexpressing WT PFKFB3 ( Fig. 6 ). The cells expressing the R131/134L mutant and those overexpressing R131/134K exhibited a significant metabolic shift from glycolysis to PPP. To be noted was the fact that the R131/134L mutant-expressing cells exhibited greater decrease in Σglycolysis values than the R131/134K mutant-expressing cells, suggesting a potent inhibitory effect of the latter mutant on the PFKFB3 activity. These results showed that the two different unmethylable mutants of PFKFB3 facilitate directional glucose utilization towards PPP. 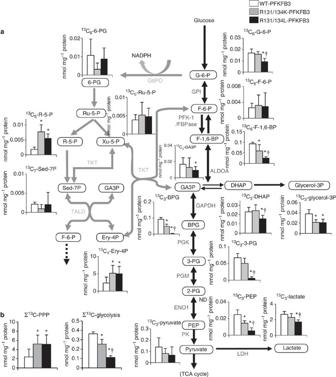Figure 6: Overexpression of unmethylable PFKFB3 mutants shifts glucose metabolism towards PPP. HEK293 cells were transfected with WT-PFKFB3, R131/134L- or R131/134K-PFKFB3 mutant. These cells were incubated with the medium containing 1 g l−1 13C6-labelled glucose for 5 min. Measurements of13C-labelled metabolites were performed by CE-MS. (a) Differences in13C-labelled metabolites in glycolysis and PPP between the cells transfected with WT-PFKFB3 (open bars), those transfected with R131/134K-PFKFB3 (grey bars) and those transfected with R131/134L-PFKFB3 (closed bars). Data are expressed as mean+s.d. (nmol mg−1protein) of six separate experiments *P<0.05 versus controls. ND, not detected. (b) The two nonmethylable mutants significantly increase PPP flux and suppress glycolysis. Differences in biotransformation of glucose in the cells carrying WT-PFKFB3 or two nonmethylable mutant: R131/134K and R131/134L. ∑13C-glycolysis and ∑13C-PPP are described inFig. 1andSupplementary Fig. 1. BPG is expressed as total sum values of 2,3-BPG and 1,3-BPG. Note that the R131/134L mutant displays greater suppression of the glycolytic flux than the R131/134K mutant (†P<0.05). Data are expressed as mean+s.d. (nmol mg−1protein) of six to seven separate experiments. *P<0.05 versus the cells carrying WT-PFKFB3. ANOVA with Fischer’s multiple comparison test was used throughout this figure. Figure 6: Overexpression of unmethylable PFKFB3 mutants shifts glucose metabolism towards PPP. HEK293 cells were transfected with WT-PFKFB3, R131/134L- or R131/134K-PFKFB3 mutant. These cells were incubated with the medium containing 1 g l −1 13 C 6 -labelled glucose for 5 min. Measurements of 13 C-labelled metabolites were performed by CE-MS. ( a ) Differences in 13 C-labelled metabolites in glycolysis and PPP between the cells transfected with WT-PFKFB3 (open bars), those transfected with R131/134K-PFKFB3 (grey bars) and those transfected with R131/134L-PFKFB3 (closed bars). Data are expressed as mean+s.d. (nmol mg −1 protein) of six separate experiments * P <0.05 versus controls. ND, not detected. ( b ) The two nonmethylable mutants significantly increase PPP flux and suppress glycolysis. Differences in biotransformation of glucose in the cells carrying WT-PFKFB3 or two nonmethylable mutant: R131/134K and R131/134L. ∑ 13 C-glycolysis and ∑ 13 C-PPP are described in Fig. 1 and Supplementary Fig. 1 . BPG is expressed as total sum values of 2,3-BPG and 1,3-BPG. Note that the R131/134L mutant displays greater suppression of the glycolytic flux than the R131/134K mutant ( † P <0.05). Data are expressed as mean+s.d. (nmol mg −1 protein) of six to seven separate experiments. * P <0.05 versus the cells carrying WT-PFKFB3. ANOVA with Fischer’s multiple comparison test was used throughout this figure. Full size image CO decreases methylated PFKFB3 to cause chemoresistance As described above, methylation levels of PFKFB3 determines the capacity of NADPH/GSH system to ameliorate oxidative stress in human monoblastic leukaemia U937 cells. We examined whether the decrease in methylated PFKFB3 serves as a switch for directional glucose metabolism towards PPP in different types of cancer cells. Human-derived HCT116 colon cancer cells and HEK293 cells were transfected with control non-targeted shRNA, or with two different forms of short hairpin RNA interference (shCBS#1 and #2). Stable CBS knockdown by shCBS decreased amounts of methylated PFKFB3 in both cell-types, while amounts of total PFKFB3 protein were unchanged ( Fig. 7a ). Maintenance of the total PFKFB3 amounts in shCBS-treated cells was not observed in those treated with the transient siCBS experiments using U937 cells ( Figs 4d and 5d ). In HCT116 cells in culture, CBS knockdown increased NADPH contents and NADPH/NADP + ratio ( Fig. 7b ), and GSH contents and GSH/GSSG ratio ( Fig. 7c ). Knocking down CBS or PRMT1 for decreasing methylated PFKFB3 significantly attenuated endogenous generation of reactive oxygen species (ROS) in the cells ( Fig. 7d ). The cells carrying control shRNA exhibited cell death in response to cisplatin in a dose-dependent manner, while those carrying shCBS exhibited significant suppression of the cisplatin sensitivity ( Fig. 7e ) that coincided with attenuating the dose-dependent augmentation of oxidative stress by cisplatin ( Fig. 7f ). The CBS knockdown in HeLa cells also increased NADPH contents and the NADPH/NADP + ratio, which coincided with ROS suppression and decreased sensitivity to cisplatin ( Supplementary Figs 9a–e ). Such a chemoresistance against cisplatin was reproduced by PRMT1 knockdown ( Supplementary Fig. 9f ), being in good agreement with a notion that a decrease in methylated PFKFB3 increases anti-oxidative capacity of cancer cells. 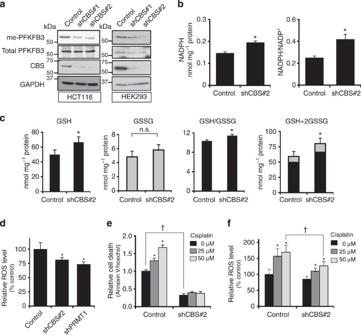Figure 7: CBS knockdown suppresses PFKFB3 methylation to cause chemoresistance. (a) Evaluations of non-overlapping shRNAs against human CBS (shCBS#1 and #2) on PFKFB3 R131/134 methylation in HCT116 (left) and HEK293 (right). Lysates were immunoblotted with anti-dimethyl-PFKFB3 (R131/134), anti-PFKFB3 and anti-CBS antibodies. The expression level of GAPDH was used as a loading control. (b) Intracellular NADPH contents and NADPH/NADP+ratio in HCT116 cells expressing shCBS#2 stably. Data indicate the mean+s.d. (n=4 independent experiments with unpaired Student’st-test). *P<0.05 versus controls. (c) Alterations in GSH, GSSG and GSH/GSSG ratio in CBS knockdown HCT116 cells. Data indicate the mean+s.d. (n=6 independent experiments; unpaired Student’st-test). *P<0.05 versus controls. n.s., not significant. (d) Suppression of intracellular ROS level in the cells silencing of CBS or PRMT1 by shRNA. Data indicate the values of relative ROS levels (mean+s.d.,n=8); *P<0.05 versus controls. (e) Effects of CBS knockdown on the toxicity of cisplatin in HCT116 cells. HCT116 cells were treated with increasing concentrations of cisplatin for 16 h. Values of relative cell death are expressed as mean+s.d. (n=4). *P<0.05 versus controls without cisplatin.†P<0.05 for shCBS#2 versus control without cisplatin. (f) Alterations in endogenous ROS levels with increasing concentrations of cisplatin in the cells carrying control or shCBS#2. Note that treatment of cisplatin upregulates intracellular ROS levels in a dose-dependent manner in the control cells, while those transfected with shCBS#2 displayed the partial suppression of cellular ROS levels. Data indicate mean+s.d. for eight separating experiments. *P<0.05 versus controls (without cisplatin).†P<0.05 for the cells transfected with shCBS#2 versus controls in the presence of 50 μM cisplatin. Statistical analysis used in (d–f) was ANOVA with Fischer’s multiple comparison test. Figure 7: CBS knockdown suppresses PFKFB3 methylation to cause chemoresistance. ( a ) Evaluations of non-overlapping shRNAs against human CBS (shCBS#1 and #2) on PFKFB3 R131/134 methylation in HCT116 (left) and HEK293 (right). Lysates were immunoblotted with anti-dimethyl-PFKFB3 (R131/134), anti-PFKFB3 and anti-CBS antibodies. The expression level of GAPDH was used as a loading control. ( b ) Intracellular NADPH contents and NADPH/NADP + ratio in HCT116 cells expressing shCBS#2 stably. Data indicate the mean+s.d. ( n =4 independent experiments with unpaired Student’s t -test). * P <0.05 versus controls. ( c ) Alterations in GSH, GSSG and GSH/GSSG ratio in CBS knockdown HCT116 cells. Data indicate the mean+s.d. ( n =6 independent experiments; unpaired Student’s t -test). * P <0.05 versus controls. n.s., not significant. ( d ) Suppression of intracellular ROS level in the cells silencing of CBS or PRMT1 by shRNA. Data indicate the values of relative ROS levels (mean+s.d., n =8); * P <0.05 versus controls. ( e ) Effects of CBS knockdown on the toxicity of cisplatin in HCT116 cells. HCT116 cells were treated with increasing concentrations of cisplatin for 16 h. Values of relative cell death are expressed as mean+s.d. ( n =4). * P <0.05 versus controls without cisplatin. † P <0.05 for shCBS#2 versus control without cisplatin. ( f ) Alterations in endogenous ROS levels with increasing concentrations of cisplatin in the cells carrying control or shCBS#2. Note that treatment of cisplatin upregulates intracellular ROS levels in a dose-dependent manner in the control cells, while those transfected with shCBS#2 displayed the partial suppression of cellular ROS levels. Data indicate mean+s.d. for eight separating experiments. * P <0.05 versus controls (without cisplatin). † P <0.05 for the cells transfected with shCBS#2 versus controls in the presence of 50 μM cisplatin. Statistical analysis used in ( d – f ) was ANOVA with Fischer’s multiple comparison test. Full size image CBS knockdown increases GSH/GSSG to stimulate tumour growth In our studies, CBS knockdown in HCT116 cells or overexpression of unmethylable R131/134K mutant in HEK293 cells significantly accelerated cell proliferation ( Supplementary Fig. 10 ), suggesting a critical role of CBS in modulating PFKFB3 methylation to enhance GSH/GSSG against oxidative stress. We therefore inquired whether CBS knockdown in HCT116 cells results in enhancement of GSH/GSSG in vivo , since increasing GSH/GSSG might help cancer proliferation so far as our recent observation showed that cancer cells undergoes increased oxygen consumption to expose themselves to oxidative stress during G2/M phase [28] . Taking advantage of quantitative imaging mass spectrometry (Q-IMS) to determine regional contents of metabolites in tumours in vivo as well as clinical relevance of transportal metastasis of colon cancer in the liver, we examined GSH and GSSG using an experimental model of xenograft transplantation of HCT116 cells in superimmunodeficient NOG mice [28] , [29] , [30] . HCT116 cells stably transfected with shCBS against two different target sequences (shCBS#1 and #2) or with non-targeted control shRNA were injected into spleens of NOG mice to induce liver metastasis. At 2 weeks after the cell transplantation in spleen, the size of tumours derived from CBS-knocked down cells was significantly greater than the non-target control shRNA-expressing tumour ( Fig. 8a ). The relative percentages of tumour occupancy of shCBS-carrying HCT116 cells in the host liver were significantly greater than the non-target control. The greatest effects of growth stimulation were seen in the shCBS#2-treated cells ( Fig. 8b ). These results are consistent with a notion that enhancement of NADPH/GSH system by CBS knockdown benefits tumour growth in vivo . So far as judged by CE-MS analyses using snap-frozen tumour-bearing liver samples, CBS knockdown significantly decreased GSSG contents, and resultantly increased the GSH/GSSG ratio in tumour-bearing liver tissues as a whole. The tissue contents of total glutathione in vivo were unchanged by shCBS#2 treatment ( Fig. 8c ). 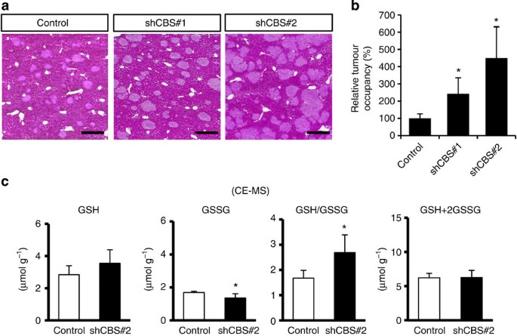Figure 8: Effects of CBS knockdown on tumour growth and tissue glutathione contents in HCT116 xenograft-bearing livers. (a) The representative pictures of hematoxylin–eosin-stained liver slices, indicating hepatic micrometastases of HCT116 xenograft. The cancer cells were expressing control or shRNA against different target sequences of CBS (shCBS#1 and #2). After 2 weeks, tumour growth is examined. Scale bar, 500 μm (b) Differences in the relative occupancy rates of metastatic tumours in the liver. Data express mean+s.d. for five separate experiments. *P<0.05 versus controls (ANOVA with Fischer’s multiple comparison test). (c) Differences in CE-MS data of reduced and oxidized glutathione contents in livers with micrometastasis of HCT116 cells carrying control (open bars) and shCBS#2 (closed bars). Data show mean+s.d. of five separate experiments. *P<0.05 versus controls. Unpaired Student’st-test was used for statistical analyses. Figure 8: Effects of CBS knockdown on tumour growth and tissue glutathione contents in HCT116 xenograft-bearing livers. ( a ) The representative pictures of hematoxylin–eosin-stained liver slices, indicating hepatic micrometastases of HCT116 xenograft. The cancer cells were expressing control or shRNA against different target sequences of CBS (shCBS#1 and #2). After 2 weeks, tumour growth is examined. Scale bar, 500 μm ( b ) Differences in the relative occupancy rates of metastatic tumours in the liver. Data express mean+s.d. for five separate experiments. * P <0.05 versus controls (ANOVA with Fischer’s multiple comparison test). ( c ) Differences in CE-MS data of reduced and oxidized glutathione contents in livers with micrometastasis of HCT116 cells carrying control (open bars) and shCBS#2 (closed bars). Data show mean+s.d. of five separate experiments. * P <0.05 versus controls. Unpaired Student’s t -test was used for statistical analyses. Full size image To further examine local contents of these metabolites in individual tumours, Q-IMS based on matrix-assisted laser desorption/ionization (MALDI) was carried out ( Fig. 9a ). As judged by imaging UDP-N-acetyl-hexosamine (UDP-HexNAc) as a tumour marker [30] , tumours derived from shCBS-transfected HCT116 cells developed the size of metastases, being consistent with the results in Fig. 8a,b . The development of tumour growth in shCBS-transfected HCT116 xenografts coincided with a decrease in regional GSSG contents ([GSSG] app in Fig. 9b ) and an increase in the ratio of [GSH] app /[GSSG] app in metastases with statistical significance. These results suggested that the increase in GSH/GSSG in HCT116-derived tumours results not only from the increasing size of metastases but also from metabolic alterations in local cancer cells forming individual tumours in vivo . 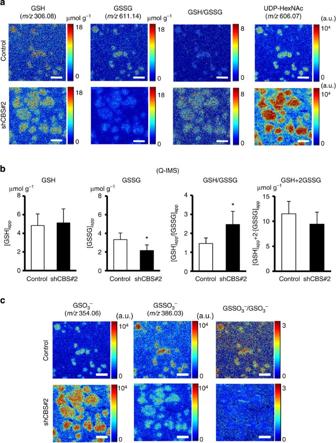Figure 9: Increased GSH/GSSG and decreased glutathione S-sulphonate in HCT116-derived tumours knocking down CBS. (a) Representative pictures of quantitative imaging mass spectrometry (Q-IMS) to determine regional contents of reduced (GSH) and oxidized glutathione (GSSG) in tumour-bearing liver. Data showed the apparent contents of GSH atm/z306.08, GSSG atm/z611.14 and [GSH]app/[GSSG]appratio. UDP-HexNAc atm/z606.07 was also visualized in the same tissue section to identify localization of HCT116-derived tumours. UDP-HexNAc was shown as a marker metabolite enriched in hepatic micrometastasis of HCT116 (ref.30). Pseudocolor bars indicate apparent contents of metabolites (μmol per gram of tissue). The ratio image of GSH/GSSG was also generated. Scale bar, 500 μm. (b) Quantitative determination of apparent contents of GSH [GSHapp], GSSG [GSSGapp], GSH/GSSG [GSHapp]/[GSSGapp] and total glutathione contents in HCT116-derived tumours. Data indicate mean+s.d. of five separate experiments. *P<0.05 versus controls (unpaired Student’st-test). (c) Representative pictures of GSO3−atm/z354.06, glutathione S-sulphonate (GSSO3−) atm/z386.03, and the ratio image of GSSO3−/GSO3−in metastatic tumours derived from HCT116 cells treated with non-targeting control shRNA and those treated with shCBS#2. The microscopic field is identical to that shown ina. Right color bar and associated numbers indicate a.u. or ratio with red and blue representing high and low amounts, respectively. Scale bar, 500 μm. Figure 9: Increased GSH/GSSG and decreased glutathione S-sulphonate in HCT116-derived tumours knocking down CBS. ( a ) Representative pictures of quantitative imaging mass spectrometry (Q-IMS) to determine regional contents of reduced (GSH) and oxidized glutathione (GSSG) in tumour-bearing liver. Data showed the apparent contents of GSH at m/z 306.08, GSSG at m/z 611.14 and [GSH] app /[GSSG] app ratio. UDP-HexNAc at m/z 606.07 was also visualized in the same tissue section to identify localization of HCT116-derived tumours. UDP-HexNAc was shown as a marker metabolite enriched in hepatic micrometastasis of HCT116 (ref. 30 ). Pseudocolor bars indicate apparent contents of metabolites (μmol per gram of tissue). The ratio image of GSH/GSSG was also generated. Scale bar, 500 μm. ( b ) Quantitative determination of apparent contents of GSH [GSH app ], GSSG [GSSG app ], GSH/GSSG [GSH app ]/[GSSG app ] and total glutathione contents in HCT116-derived tumours. Data indicate mean+s.d. of five separate experiments. * P <0.05 versus controls (unpaired Student’s t -test). ( c ) Representative pictures of GSO 3 − at m/z 354.06, glutathione S-sulphonate (GSSO 3 − ) at m/z 386.03, and the ratio image of GSSO 3 − /GSO 3 − in metastatic tumours derived from HCT116 cells treated with non-targeting control shRNA and those treated with shCBS#2. The microscopic field is identical to that shown in a . Right color bar and associated numbers indicate a.u. or ratio with red and blue representing high and low amounts, respectively. Scale bar, 500 μm. Full size image Recent observations have shown that CBS might participate in the regulation of cancer proliferation and chemoresistance through mechanisms involving H 2 S/HS − : some studies suggest stimulatory effects while others suggest inhibitory effects on proliferation [31] , [32] , [33] , indicating conflicting results of roles of H 2 S/HS − . Although direct visualization of H 2 S/HS − was technically difficult in vivo , we examined whether CBS knockdown in HCT116 cells alters glutathione S-sulphonate (GSSO 3 − ), a terminal oxidized product yielded by H 2 S/HS − from GSH and GSSG under atmospheric MALDI condition, respectively ( Supplementary Fig. 11 ). This is because of the fact that thiol-containing compounds are automatically oxidized by ionization under atmospheric conditions in vitro [34] ; GSH and glutathione persulphide (GSS − ), which is generated through the reaction of H 2 S/HS − with GSH, are oxidized and detected as glutathione sulphonate (GSO 3 − ) at m/z 354.06, and GSSO 3 − at m/z 386.03 as stable endproducts, respectively. Namely, atmospheric MALDI detection of GSSO 3 − might serve as an indirect index of endogenous H 2 S/HS − generation. According to the previous method showing that the mixture of GSSG with NaHS generates GSSH [35] , we prepared the standard persulfide solution and exposed it to MALDI procedure to analyse the profile by tandem MS. Experiments in vitro showed generation of GSS − and GSSO 3 − from GSH in the presence of NaHS ( Supplementary Fig. 11a,b ). These results indicate that neither GSS − nor GSSO 3 − is generated from GSH without NaHS. GSSO 3 − was also generated from GSSG in the presence of NaHS ( Supplementary Fig. 11c ). Tandem MS profiles of the peak at m/z 386.03 (GSSO 3 − ) and 354.06 (GSO 3 − ) detected in the HCT116 xenograft-derived tumour in vivo ( Supplementary Fig. 11e,g ) were consistent with those detected in the NaHS-derived persulfide solution containing GSO 3 − or GSSO 3 − , respectively ( Supplementary Fig. 11d–g ). These results suggested that GSSO 3 − as the GSS − -derived oxidized product is detectable in the tumour-bearing liver in vivo under MALDI-MS analyses. Based on these data, we compared differences in GSO 3 − and GSSO 3 − between cancer xenografts treated with non-target shRNA and shCBS#2. As seen in Fig. 9c that indicated the same microscopic field shown in Fig. 9a , HCT116-derived metastatic tumours exhibited strong MS signals of GSO 3 − and GSSO 3 − compared with the parenchymal region in the same tissue section. HCT116-derived tumours indicated greater GSO 3 − signals with smaller GSSO 3 − signals than those treated with non-target control shRNA. The ratio image of GSSO 3 − /GSO 3 − suggested that endogenous GSS − generation appears smaller in tumours derived from the shCBS-transfected HCT116 cells than in those derived from the control HCT116 cells ( Fig. 9c ). These results suggested that endogenous H 2 S/HS − generation is smaller in the shCBS-treated xenografts in vivo , implicating a role of CBS in the cancer cells for endogenous H 2 S/HS − generation in situ . We have shown a novel molecular mechanism by which CO acts as a regulator for the directional biotransformation of glucose through the arginine methylation of PFKFB3. Metabolome analyses revealed that effects of the HO-1 induction in U937 cells on a shift of glucose biotransformation towards PPP flux were approximately threefold greater than the basal flux, while those on suppression of glycolysis were ~50% of the basal control ( Fig. 1 ). Mechanisms appear to involve CO-dependent inhibition of CBS and subsequent alterations of remethylation metabolism that resultantly suppress PFKFB3 methylation. Furthermore, the results provide evidence for the first example indicating a crucial role of site-specific asymmetric dimethylarginine modification of the carbohydrate-metabolizing enzyme in modulating directional biotransformation of glucose towards PPP in the cells. PFKFBs are bifunctional enzymes that generate and degrade F-2,6-BP, a potent allosteric effector of PFK-1 (ref. 36 ). Previous studies showed that the expression levels of two inducible isoforms of PFKFBs play important roles in rapid proliferation of cancer cells [37] , [38] , [39] . One is a PFKFB variant, TIGAR ( T p53- i nduced g lycolysis and a poptosis r egulator); because of its absence of kinase activity, this variant has been shown to protect cancer cells against oxidative stress through PPP-dependent NADPH generation in glioma and multiple myeloma cells [40] , [41] , [42] . Another is PFKFB3, the isozyme lacking phosphatase activities, which is upregulated by hypoxia and AMPK signalling [43] , [44] . PFKFB3 possesses higher kinase activity for production of F-2,6-BP, expressing predominantly in embryonic cells and cancer cells [36] , [43] . Considering the structural proximity of the R131/R134 region of PFKFB3 to other functional domains of the enzyme ( Supplementary Fig. 6 ), the current results provided evidence for critical roles of the R131/134-specific methylation for regulating sensitivity to K142-specific polyubiquitination and enzymatic ability to generate F-2,6-BP. First, recent studies have revealed that polyubiquitination of PFKFB3 is a critical step leading to degradation through the E3 ubiquitin ligase APC/C-cdh1 (ref. 26 ), although stabilizing mechanisms for PFKFB3 remain largely unknown. Considering that the R131/134 region is spatially close to K142, the target residue for polyubiquitination ( Fig. 3d and Supplementary Fig. 6 ), it is not unreasonable to suggest that methylation of these arginine residues contributes to constitutive PFKFB3 stabilization in cancer cells. Second, previous studies showed that R133, another arginine residue proximal to methylated arginine residues (R131/134) on the same helix, is able to interact with fructose-6-phosphate (F-6-P), the substrate of PFKFB3 with the covalent bond [45] . The current observation that R131/134K mutant-transfected cells displayed lower PFKFB3 activity than the WT-transfected cells ( Fig. 5f ) is in good agreement with a hypothesis that R131/134 methylation facilitates F-6-P binding to the enzyme. Of interest is that the cells overexpressing the R131/134L mutant displayed more potent suppression of glycolytic conversion than those overexpressing the R131/134K mutant; these results suggest that interference with PFKFB3 methylation by the double R/L-mutant results in downregulation of glycolysis ( Fig. 6 ), presumably because of its potent inhibitory action on the PFKFB3 activity. A potential steric effect of the lysine residue of the mutant PFKFB3 on the enzyme activity should further been examined. Collectively, these observations are consistent with a notion that asymmetric dimethylarginine modification of R131/134 does not only interfere with the recruitment of ubiquitin ligase for the enzyme degradation but also maintain glycolysis in cancer cells. There are several therapeutic strategies targeting PFKFB3 for cancer treatment [46] , [47] . The current results shed light on a novel molecular basis for controlling activities and degradation of PFKFB3 through modulation of methylation that might benefit for the refinement of anti-cancer therapeutics. In microenvironments in vivo , cancer cells have been thought to be exposed to incomplete oxygenation that paradoxically causes oxidative stress through multiple mechanisms involving suppressed mitochondrial electron transfer and increased NADH (refs 48 , 49 ). Accumulation of inflammatory cells surrounding tumours and exposure to therapeutic interventions such as radiation and anti-cancer reagents serve as other resources of oxidative stress in vivo [27] , [50] . Under proliferative conditions, cancer cells in G2/M phase exhibit greater extents of O 2 consumption, mitochondrial respiration and ROS generation than those in G1 phase, suggesting that the cells are exposed to oxidative stress periodically during the proliferative cycle [28] . To protect against several resources of oxidative stress, cancer cells turned out to accumulate relatively high concentrations of GSH versus GSSG in vitro and in vivo [30] , [51] , [52] . Considering metabolic pathways in non-malignant cells under physiological conditions, CO-dependent CBS inhibition might downregulate trans-sulphuration pathway to suppress glutathione synthesis. As seen in experiments in U937 cells, CO application or HO-1 induction by haemin actually decreased total amounts of glutathione ( Fig. 5c ). However, such an effect was surpassed by the potency of CO to shift towards PPP and to increase NADPH and the GSH/GSSG ratio. In HCT116 cells, which highly express CD44 variant and possess the ability to uptake cystine from extracellular space through glutamate–cystine transporter (xCT) [53] , the cultured cells ( Fig. 7 ) as well as xenograft tumours in vivo ( Figs 8 and 9 ) appear to compensate glutathione synthesis, even under CBS knockdown conditions. Actually, HCT116 cells undergoing CBS knockdown increased GSH/GSSG without decreasing total glutathione contents both in vitro and in vivo ( Figs 7 , 8 , 9 ), supporting the aforementioned notion. In summary, cancer cells appear to utilize two discernible forms of PFKFB3, an asymmetrically di-methylated form that increases F-2,6-BP for PFK-1 activation and an unmethylated form that causes a shift of glucose biotransformation directionally towards PPP ( Fig. 10 ). Under exposure to anti-cancer reagents, radiation therapy, oxidative stress or prolonged hypoxia ( Fig. 10 and Supplementary Fig. 12 ), cancer cells upregulate HO-1/CO system. Under these circumstances, the cancer cells utilize CBS to suppress PFKFB3 methylation to ensure synthesis of reducing equivalents such as NADPH and GSH for survival at an expense of glycolytic energy management. The CO/CBS-assisted signalling system does not only serve as a switch for decreasing methylated PFKFB3 but also accounts for a mechanism for H 2 S/HS − -mediated bioregulation [5] , [14] . So far as judged by a decrease in the GSSO 3 − /GSO 3 − ratio in CBS knockdown tumours in vivo , endogenous HS − suppression is likely to coincide with cancer proliferation. However, by developing a reliable quantitative method for short-lived HS − and persulphide metabolites to investigate biological actions of these species [54] , roles of tumour-derived H 2 S/HS − for cancer survival should carefully be examined in vivo . Mechanisms for regulating tenuous balance between methylated and unmethylated forms of PFKFB3 for cancer survival deserve further studies, provided that therapeutic interventions targeting the methylation switch lead to the suppression of cancer proliferation in vivo . 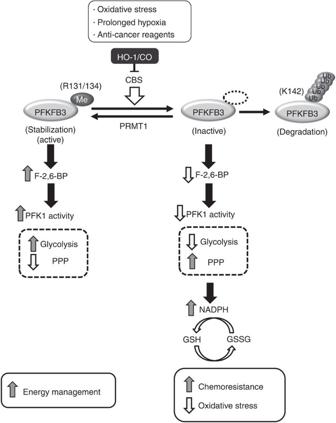Figure 10: A schematic model for the regulation of directional glucose metabolism via PFKFB3 methylation by CO/CBS system. Stress-induced CO production suppresses CBS activity, results in a decrease in methylated PFKFB3. Arginine methylation of PFKFB3 (R131/134) stabilizes the enzyme to enhance glycolysis through the augmentation of F-2,6-BP, an allosteric activator of PFK1. On the other hand, unmethylated PFKFB3 is prone to polyubiquitination (K142), leading to the ubiquitin/proteasome pathway-dependent degradation of the enzymes. As a result, methylated PFKFB3 is decreased to shift glucose biotransformation towards PPP. Acceleration of PPP increases cellular NADPH amounts, providing a reducing equivalent for glutathione that benefits enhancement of chemoresistance and/or amelioration of oxidative stress during proliferation of cancer cells. Figure 10: A schematic model for the regulation of directional glucose metabolism via PFKFB3 methylation by CO/CBS system. Stress-induced CO production suppresses CBS activity, results in a decrease in methylated PFKFB3. Arginine methylation of PFKFB3 (R131/134) stabilizes the enzyme to enhance glycolysis through the augmentation of F-2,6-BP, an allosteric activator of PFK1. On the other hand, unmethylated PFKFB3 is prone to polyubiquitination (K142), leading to the ubiquitin/proteasome pathway-dependent degradation of the enzymes. As a result, methylated PFKFB3 is decreased to shift glucose biotransformation towards PPP. Acceleration of PPP increases cellular NADPH amounts, providing a reducing equivalent for glutathione that benefits enhancement of chemoresistance and/or amelioration of oxidative stress during proliferation of cancer cells. Full size image Antibodies and chemicals All experiments requiring gene recombination and transfection in this study were carried out in accordance with the institutional guidelines of Keio University School of Medicine. The primary antibody used were anti-PFKFB3 mouse monoclonal (H00005209-M08, Abnova, Taipei, Taiwan; 3,000 × dilution), anti-PFKFB3 rabbit polyclonal (H00005209-D01P, Abnova; 3,000 × dilution), anti-FLAG M2 mouse monoclonal (A9469, SIGMA-Aldrich, St Louis, MO; 100,000 × dilution), anti-V5 HRP conjugate (46-0708, Invitrogen, Carlsbad, CA; 5,000 × dilution), anti-CBS mouse monoclonal (H00000875-M01, Abnova; 7,000 × dilution), anti-PRMT1 rabbit polyclonal (07-404, Millipore, Billerica, MA; 5,000 × dilution), anti-PRMT4 (also known as CARM1) rabbit polyclonal (07-080, Millipore; 5,000 × dilution), anti-HO-1 rabbit polyclonal (SPA-896; Assay Designs, Farmingdale, NY; 5,000 × dilution), anti-GAPDH goat polyclonal (sc-20357, Santa Cruz Biotechnology, Inc., Santa Cruz, CA; 10,000 × dilution), anti-Cdh1 mouse monoclonal (NBP2-19018, NOVUS biologicals, Littleton, CO; 5,000 × dilution). A rabbit polyclonal antibody for asymmetrically di-methylated R131/R134 PFKFB3 was generated by SIGMA-Aldrich Japan (Ishikari, Japan; 5,000 × dilution). The antisera were obtained by immunizing with the methylated peptide as follows: IAVFDATNTTR(ADMA)ERR(ADMA)HMI. The sera were purified over peptide-affinity column. The adenosine dialdehyde (AdOx, A7154), an inhibitor of S-adenosylhomonocysteine hydrolase (SAHH), haemin (H-5533), MG132 (C2211), puromycin (P7255) and actinomycin D (A1410) were purchased from SIGMA-Aldrich. G418 is purchased from Calbiochem (345810, Darmstadt, Germany). Isopropyl-β-D-thiogalactopyranoside (IPTG, 09-0514) was purchased from WAKO Pure Chemical Industries (Osaka, Japan). Ruthenium (III) chloride and CO-releasing molecule-2 (CORM-2) were purchased from SIGMA-aldorich as described previously [15] . Chromium (III) mesoprotoporphyrin IX (CrMP) chloride was purchased from Frontier Scientific Inc (P40185, Logan, UT). Uncropped scans of representative western blots used in the current study are shown in Supplementary Fig. 13 . Cell culture U937 cells were obtained from the American Type Culture Collection (ATCC), and cultured in RPMI1640 (Invitrogen) supplemented with 10% FBS (SIGMA-Aldrich), penicillin–streptomycin (Invitrogen). Stable transfectants of WT HO-1 or mutant HO-1 (H25A) in U937 cells were established as described previously [25] . Adherent cell lines, HEK293, HeLa and HCT116 cells were cultured with DMEM (Invitrogen) containing with 10% FBS, penicillin streptomycin. When necessary, PBS is saturated with 100% CO gas (Nippon MEGACARE, Tokyo, Japan) for 20 min on ice. CO-saturated PBS (around 1 mM) was diluted with RPMI1640 to 5 μM (final concentration). For haemin treatment, the cells were treated with 25 μM haemin for 6 h. The cells (5 × 10 6 ) treated with AdOx for 16 h, or 5 μM CO for 30 min or 25 μM haemin for 6 h were washed with PBS twice, and were then frozen in liquid nitrogen. Determination of PFK-1 activity and F-2,6-BP contents PFK-1-specific activities were measured using a coupled spectrophotometric assay by monitoring the rate of F-1,6-BP formation from F-6-P and ATP [43] . Approximately 1 × 10 7 cells were sonicated in 0.2 ml of lysis buffer containing 50 mM Tris-HCl (pH 8.0), 10 mM dithiothreitol (DTT), 1 mM EDTA, 1 mM EGTA, 0.02% phenylmethylsulfonyl fluoride and centrifuged at 20,000 g for 30 min, then the supernatants were used for the assay. Relative PFK-1 activities were expressed as the ratio of PFK-1 activity obtained from control lysate derived from non-treated cells as 100% activity. F-2,6-BP was determined in supernatants by its ability to activate pyrophosphate-dependent PFK-1 (F2258, SIGMA-Aldorich) from potato tubers according to the previous method [55] . Determination of intracellular metabolites U937 cells (2 × 10 7 cells per 100-mm dish) were used for the determination of 13 C 6 -labelled glycolytic metabolites. Control or 25 μM haemin-treated cells (for 6 h) were inoculated with the RPMI1640 medium containing 2 g l −1 13 C 6 -labelled glucose (389374, SIGMA-Aldrich: ISOTEC). The cells were then harvested for 5 min with the 13 C 6 -labelled glucose-containing medium. Subsequently, the cells were washed with PBS twice, and were followed by washing with 5% ( w / v ) mannitol twice to be frozen quickly by liquid nitrogen. Metabolome analyses in the cells transfected with WT- and R131/134L-PFKFB3 mutant were performed using HEK293 cells. Transfected cells (~2 × 10 7 cells per 100-mm dish) were incubated with DMEM, containing 13 C 6 -labelled glucose (1 g/l) for 5 min, an sufficient period of time to identify 13 C 6 -glucose conversion to the downstream intermediates belonging to PPP and glycolysis. Following the rinse with PBS, the cells were washed with 5% mannitol, and then frozen by liquid nitrogen. Metabolites were extracted from cells with a solvent composed of methanol, distilled water and chloroform (methanol: water: chloroform=1:0.5:1 ( v / v / v )). After centrifugation at 20,000 g at 4 °C for 15 min, the supernatants were filtered through 5-kDa cutoff filter (Millipore). Metabolites including those that had at least one 13 C atom in the filtrate were analysed by using an Agilent CE Capillary Electrophoresis System equipped with an Agilent 1100 series MSD mass spectrometer [28] , [56] . Labelled metabolites containing at least one 13 C atom in a molecule were collectively indicated as 13 C-labelled forms. For fluxome analyses, Σglycolysis was calculated as the sum of intermediates of glycolysis (glucose-6-phosphate+fructose-6-phosphate+fructose-1,6-bisphosphate+glyceraldehyde-3-phosphate+dihydroxyacetone phosphate+bisphosphoglycerate+3-phosphoglycerate+2-phosphoglycerate+phosphoenolpyruvate), while ΣPPP was the sum values of the metabolites in PPP (glucose-6-phosphate+fructose-6-phosphate+6-phosphogluconate+ribulose-5-phosphate+ribose-5-phosphate+sedoheptulose-7-phosphate+erythrose-4-phosphate+glyceraldehyde-3-phosphate). The energy charge (EC) was calculated using the values for ATP, ADP and AMP, as the following. The determinations of sulfur-containing amino acids were carried out with API3000 LC-MS [2] systems (Applied Biosystems) equipped with a turbo ion spray source as described previously [15] . In brief, U937 cells (1 × 10 6 cells) were treated with 5 μM CO for 30 min or with 25 μM haemin for 6 h, and were then washed with PBS twice and frozen quickly by liquid nitrogen. For the determination of 15 N-labelled cystathionine, The CBS-silencing U937 cells (1 × 10 7 cells) treated with 100 μM Ruthenium (III) chloride (RuCl 3 ) or CORM-2-treated U937 were incubated with RPMI1640 medium containing 75 mg l −1 15 N-labelled methionine (609242, SIGMA-Aldrich: ISOTEC) for 5 min. The metabolites were extracted with methanol/chloroform method. After centrifugation at 20,000 g at 4 °C for 15 min, the supernatants were filtered through a 5-kDa cutoff filter (Millipore); to examine the metabolites in the filtrate it was analysed by using an Agilent CE Capillary Electrophoresis System equipped with an Agilent 1100 series MSD mass spectrometer [12] , [56] . Cellular NADPH contents were determined by colorimetric determination method using NADP/NADPH determination kit according to the manufacturer’s manual (Biovision, Milpitas, CA). The U937, HEK293, HeLa and HCT116 cells were obtained from ATCC, and 5 × 10 6 cells for each cell lines were used for the NADPH determination. Values were normalized by the amount of total protein. Intracellular reduced and oxidized glutathione contents were determined with CoulArray multi-electrode array detector system (Model 5600A; ESA Inc, Chelmsford, MA) [15] , [57] . Briefly, 1 × 10 7 cells were homogenized in the extraction buffer (10% trichloroacetate, 100 μM Diethylenetriaminepentaacetic dianhydride (DTPA)) with sonications to obtain cellular homogenates. The homogenates were centrifuged at 16,000 g for 10 min at 4 °C, and the supernatants were filtrated through an Ultrafree-MC filter (0.45 μm, Durapore PVDF, Millipore). Samples were separated on a reversed-phase C18 column (4.6 mm × 250 mm, LMS, Tokyo, Japan) by acetonitrile gradient elution, and GSH/GSSG glutathione were detected with a CoulArray detector. Values were normalized by the amount of total protein. Raw data of metabolomics for Figs 1 and 6 are shown in Supplementary Tables 3 and 4 , respectively. Plasmid constructions and site-directed mutagenesis An expression vector of PFKFB3 was constructed as follows: the cDNA containing the coding region of human PFKFB3 was amplified with the primers described in Supplementary Table 1 , and then subcloned into pENTR-D vector (Invitrogen). The insert was converted into N-terminal GST-tagged (for the bacterial expression) and N-terminal 3xFLAG-tagged expression vector (for the expression in mammalian cells) with GATEWAY conversion system. For the construction of truncated mutants of PFKFB3, primers were used as shown in Supplementary Table 1 . The truncated fragments were ligated into BamHI/XhoI site of pGEX-6P vector (GE healthcare, Amersham, UK). Site-directed mutagenesis is carried out with KOD plus mutagenesis kit (TOYOBO, Osaka, Japan) according to the manufacturer’s manual. Primers carrying mutation of human PFKFB3 (R131K, R133K, R134K, R131/134K, R131/134L, and K142A) were described also in Supplementary Table 1 . The mammalian expression vectors for human PRMT1 and PRMT4 were constructed as follows: human PRMT1 and PRMT4 cDNA fragments were amplified with primers described in Supplementary Table 1 . Each fragment was subcloned into pENTR-D vector. Using GATEWAY system, the entry vectors carrying human PRMT1 and CARM1 were recombinated with N-terminal 3xFLAG-tagged vector or C-terminal V5-tagged vector, respectively. Plasmid and siRNA/shRNA transfection Plasmid DNA transfection into HEK293 cells was performed with Lipofectamine LTX (Invitrogen). The 4-μg plasmid DNA was transfected into six-well-plated cells (1 × 10 6 cells) according to the manufacturer’s instruction. For the construction of 3xFLAG tag-fused human PFKFB3 (WT or R131/134K) stable expression lines, the transfected cells were selected with G418 (50 μg ml −1 ) for 2 weeks. For gene-silencing experiments with siRNA for human CBS and Cdh1, siGENOME SMARTpool sets, containing siRNA mixture of four different sequences for the target genes were purchased from Dharmacon, Inc. (Lafayette, CO). The siRNA oligonucleotides targeted for human PFKFB3, PFKFB4, PRMT1 and PRMT4 were purchased from SIGMA-Aldrich. For the negative control, siRNA oligonucleotides with scrambled sequences were used (MISSION siRNA Universal Negative control#1, SIC-001, SIGMA-Aldrich). These oligonucleotides were transfected with nucleofector II instrument (Lonza Inc, Allendale, NJ) into the U937 cells [15] . Briefly, the cells were harvested for 48 h after the siRNA transfection. For the construction of stable expression systems, shRNA vectors against human PRMT1 and human CBS were purchased from Open Biosystems (Lafayette, CO). As a negative control, GIPZ Non-silencing Lentiviral shRNA Control vector (Open Biosystems, RHS4346) was used. The transfected cells were selected by puromycin (15 μg per ml of the medium) for 2 weeks. The sequences of siRNA and shRNA used throughout all studies were listed in Supplementary Table 2 . Purification of recombinant proteins Human recombinant PRMTs (PRMT1, 3–8) and PFKFB3 (WT and each mutant) proteins were constructed using E.coli expression system as follows: nucleotide sequences of primers for the construction of PRMTs are listed in Supplementary Table 1 . Each PCR fragment was subcloned into pENTR-D vector, followed by conversion into N-terminal GST-tagged vector, pDEST15 (Invitrogen), using GATEWAY conversion system. The coding region of human PFKFB3 was subcloned into pGEX-6P, bacterial expression vector as described above. The plasmids were transformed into E.coli BL21 strain. The transformed cells were cultured at 27 °C for 16 h with 1-l LB medium after the administration of 0.1 mM IPTG. After collecting cells by centrifugation, the cells were sonicated in PBS for 10 min on ice. Lysates were resolved by centrifugation and loaded onto GSTrap column (GE healthcare). After washing with PBS twice, GST-fusion proteins were eluted with elution buffer (50 mM Tris-HCl; pH7.8, 10 mM glutathione), and subsequently dialyzed with PBS. The purification efficiency was examined by Coomassie Brilliant Blue staining. In vitro methylation assay For in vitro methylation assay, recombinant GST-PFKFB3 (WT or each mutants, 2 μg each) was incubated with GST-PRMT1, 3–8 (2 μg each) in PBS, containing 0.5 mM DTT, 1.65 μCi S-adenosyl-L-[methyl- 3 H] methionine (MP biomedicals, Santa Ana, CA), and glutathione sepharose (GE healthcare) at 37 °C for 2 h. The eluted products were separated by SDS-PAGE and subsequently analysed by Coomassie Brilliant Blue staining. The radioactive signals (exposure for 24 h) were analysed using a FUJIX Bio-Imaging Analyser BAS2500 (Fuji Photo Film, Tokyo, Japan). The uncropped gel images used in this assay are shown in Supplementary Fig. 13 . Detection of PFKFB3 polyubiquitination Endogenous ubiquitinated proteins in U937 cells were enriched by Ubiquitin Enrichment kit (Thermo Fisher Scientific, Waltham, MA) according to the manufacturer’s instructions. In brief, whole-cell extracts (1 mg) were incubated with polyubiquitin affinity resin for 4 h at 4 °C. Then, the resin was washed with TBS three times, followed by elution with 1 × sample buffer. The eluted ubiquitinated proteins were separated by SDS-PAGE, and then immunoblotting was performed with anti-PFKFB3 polyclonal antibody. To detect PFKFB3 polyubiquitination, HEK293 cells transfected with FLAG-tagged WT PFKFB3 (WT) or K142A mutant PFKFB3 were used. To examine the effects of HO-1/CO-mediated arginine methylation of PFKFB3 on polyubiqutination levels of the enzyme, the cells were treated with 25 μM haemin for 6 h or co-transfected with human PRMT1. The cell lysates (250 μg) were immunoprecipitated with anti-FLAG antibody for 4 h at 4 °C. The immunoprecipitates were analysed by SDS-PAGE, and followed by immunoblotting with anti-ubiquitin antibody (Thermo Fisher Scientific; 1,000x dilution). The whole-cell extracts were analysed with anti-FLAG, anti-HO-1 and anti-GAPDH antibodies as input. Cell proliferation assay The cells were seeded in six-well plates (5 × 10 4 cells per well), and cell numbers were counted every 24 h over a 2–5-day period. Accurate cell number was measured every 24 h using a Countess automated cell counter analyser (Invitrogen). Cell viability assay and human-derived cancer xenografts Vulnerability of U937, HCT116 and HeLa cells to H 2 O 2 or cisplatin was examined by APOPercentage apoptosis assay kit (Biocolor Ltd, Co Antrim, UK) or by Cell-based Annexin V-FITC kit (Cayman chemical, Ann Arbor, MI). All animal experiments were carried out in accordance with the guidelines of Experimental Animal Committee of Keio University School of Medicine. Human colon cancer (HCT116) cells were transfected stably with non-targeting shRNA or shRNA-targeting CBS were injected into the spleen of superimmunodeficient male NOG (NOD/Shi-scid/IL-2R γnull ) mice aging at 12–16 weeks [28] , [29] , [30] . In these experiments, 1 × 10 6 HCT116 cells were injected into the spleen. Two weeks after transplantation, liver lobules of the mice fasted for 17 h were excised under sevoflurane anaesthesia and snap-frozen with liquid nitrogen. To examine tumour occupancy, 5-μm thick cryosections were stained with hematoxylin and eosin (H&E), serving as resources of microscopic images for calculating tumour occupancy rate with Image J software. Quantitative imaging mass spectrometry Using snap-frozen tissues collected from the non-targeting control- or shCBS-transfected HCT116 cell-derived tumour-bearing livers, Q-IMS was carried out according to our previous methods [28] , [30] . For Q-IMS, 5 mg ml −1 9-aminoacridine (Merck Schucardt, Hohenbrunn, Germany) in 80% ethanol solution as matrix was sprayed over the 5-μm thick liver sections that were thaw-mounted on ITO-coated glass slides (Bruker Daltonik GmbH, Bremen, Germany). Using MALDI IT-TOF mass spectrometer (Shimadzu Corp., Kyoto, Japan), we acquired the data in the negative ion mode with the scanning mass range from m/z 304.0 to 670 according to our previous methods [30] . After selecting the region of interests by light observations, a series of repeated laser irradiation at 100 times per spot was performed at 10-μm intervals at 250 × 250 spots, giving 62,500 data points in total for each scan. Averaged spectra from each region of interest were generated and statistically analysed by house-made software SIMtools (Shimadzu Imaging Mass spectrometry toolbox for MATLAB). By CE-MS analysis, we measured the concentrations of reduced and oxidized glutathione in a portion of tumour-bearing liver tissues that was adjacent to the corresponding IMS section according to our previous method [12] , [28] , [58] . Then, the apparent contents of metabolites in the tumour region were calibrated as described previously [30] . In brief, to calculate the apparent contents in tumour regions in tumour-bearing livers ([ C Tumor ] app ), the following equations were used after calculation of tumour occupancy rate ( O Tumor ) in each liver with H&E-stained sections: I Tumor , I Liver and I Average are MALDI signal intensities measured in regions of tumour metastases, liver parenchyma and the whole-tissue section, respectively. O Tumor and O Liver are the percentage areas of tumour regions and liver parenchyma, respectively. In order to calculate the values of [ C Tumor ] app , we used the equation (2) from five sets of IMS data paired with CE-MS data from five mice in each group. To construct an ion-content map, MALDI-MS data was converted to analyse format, a common multidimensional biomedical imaging format file that contains MALDI signal intensity at each pixel Ii, and equation (3) was used to calculate the apparent content of metabolites of interest at each pixel ‘ i ’ ( Ci ). Visualization of glutathione S-sulphonate (GSSO 3 − ) in tumours CBS is a hydrogen sulphide-generating enzyme that might help generation of persulphide compounds in vivo . In order to detect them in the tumour-bearing livers of NOG mice, the following experiments were carried out using MALDI-MS analyses. Reduced and oxidized glutathione and sodium hydrosulphide were purchased from SIGMA-Aldrich. 9-aminoacridine (Merck Schucardt, Hohenbrunn, Germany) was used as a matrix for negative-mode mass spectrometry. Mass spectrometric analyses and tandem MS analyses were conducted by using an atmospheric pressure matrix-assisted laser desorption/ionization ion trap time-of-flight mass spectrometer (Shimadzu, Kyoto Japan). The standard of GSSH was generated by mixing of 10 mM sodium hydrosulfide with equimolar GSH or GSSG solution and incubation at 37 °C for 15 min as described [35] . Immediately after the GSSH-generating reaction, GSSH-containing solution was mixed with 9-AA solution and spotted on stainless steel plate for MALDI-MS analyses. Negative-mode MALDI-MS analyses were conducted at appropriate laser energy and analysing conditions. Mass spectra were obtained by averaging 100,000 consecutive laser shots. Since thiol-containing compounds are automatically oxidized by ionization in atmospheric condition [34] , GSSH and GSH were oxidized and detected as glutathione S-sulphonate (GSSO 3 − ) at m/z 386.03 and glutathione sulphonate (GSO 3 − ) at m/z 354.06, respectively. To annotate the peaks at m/z 386.03 and m/z 354.06 acquired from colon cancer xenograft tissue section, tandem mass spectra were compared with those from chemically generated GSH and GSSH samples ( Supplementary Fig. 11d–f ). In order to visualize GSO 3 − and GSSO 3 − , we did not calculate [C CE-MS ] and Ci, because their generation rates are different between CE-MS and MALDI imaging. The data of GSO 3 − and GSSO 3 − were visualized by IMS according to the intensities of their mass peaks ( Fig. 9c ). Statistical analysis All quantitative results are presented as the mean±s.d. of independent experiments. Statistical differences in comparison to the control group were analysed by Student’s t -test. For experiments with multiple comparisons, data were first analysed by analysis of variance (ANOVA) with Fisher’s least significant difference. P <0.05 was considered statistically significant. How to cite this article: Yamamoto, T. et al. Reduced methylation of PFKFB3 in cancer cells shunts glucose towards the pentose phosphate pathway. Nat. Commun. 5:3480 doi: 10.1038/ncomms4480 (2014).